Giant electrode effect on tunnelling electroresistance in ferroelectric tunnel junctions Among recently discovered ferroelectricity-related phenomena, the tunnelling electroresistance (TER) effect in ferroelectric tunnel junctions (FTJs) has been attracting rapidly increasing attention owing to the emerging possibilities of non-volatile memory, logic and neuromorphic computing applications of these quantum nanostructures. Despite recent advances in experimental and theoretical studies of FTJs, many questions concerning their electrical behaviour still remain open. In particular, the role of ferroelectric/electrode interfaces and the separation of the ferroelectric-driven TER effect from electrochemical (‘redox’-based) resistance-switching effects have to be clarified. Here we report the results of a comprehensive study of epitaxial junctions comprising BaTiO 3 barrier, La 0.7 Sr 0.3 MnO 3 bottom electrode and Au or Cu top electrodes. Our results demonstrate a giant electrode effect on the TER of these asymmetric FTJs. The revealed phenomena are attributed to the microscopic interfacial effect of ferroelectric origin, which is supported by the observation of redox-based resistance switching at much higher voltages. Ferroic nanostructures comprising materials such as ferromagnets and ferroelectrics and involving components with different levels of conductivity (metals, semiconductors and insulators) represent an important class of heterostructures that are very promising for applications in advanced electronic devices [1] , [2] . Indeed, the presence of order parameters in these nanostructures renders possible to switch their electrical resistances by external stimuli, which opens the way for memory, logic and neuromorphic computing applications [2] , [3] , [4] . Remarkably, in layered heterostructures, where insulating layers have the thickness of a few nanometres only, the quantum mechanical electron tunnelling becomes the dominant conduction mechanism. A prominent example of such quantum nanostructures is a magnetic tunnel junction, where two ferromagnetic electrodes are separated by an ultrathin insulating layer acting as a potential barrier [5] , [6] , [7] , [8] , [9] . Another promising quantum nanostructure has the form of a ferroelectric tunnel junction (FTJ), where the tunnel barrier is made of a ferroelectric material [10] , [11] . FTJs attracted considerable attention since the theoretical prediction of their hysteretic current–voltage ( I–V ) characteristics and tunnelling electroresistance (TER) effect in 2005 (refs 12 , 13 ). It was shown that polarization reversal in the ferroelectric barrier may give rise to a strong change in the junction’s resistance, leading to the existence of two stable resistive states. The experimental realization of FTJs, however, is a difficult task, given that it requires the growth of ferroelectric nanolayers retaining switchable spontaneous polarization at a thickness of just a few unit cells. Nevertheless, high-quality epitaxial films grown on suitable substrates were found to possess necessary ferroelectric properties even at nanoscale thicknesses [14] , [15] , [16] , [17] , [18] , which may be attributed to the enhancement of the out-of-plane polarization by substrate-induced lattice strains [19] and the elastic stabilization of a single-domain state [20] . Based on these advancements, various FTJs have recently been successfully fabricated and the TER effect was revealed experimentally and confirmed theoretically [21] , [22] , [23] , [24] , [25] , [26] , [27] , [28] , [29] , [30] , [31] . Moreover, the functioning of solid-state memories based on FTJs has been demonstrated [3] , [32] and the memristive behaviour with resistance variations exceeding two orders of magnitude was observed for FTJs with the BaTiO 3 (BTO) barrier [32] , [33] . At the same time, multiferroic tunnel junctions, combining ferromagnetic electrodes with a ferroelectric barrier, were found to display four resistance states [21] , [24] and the ability to electrically switch the spin polarization [34] . These properties are promising for high-density memory and spintronic applications of such junctions. The choice of electrode materials, due to different screening and chemical properties at the interface, seems to have pronounced influence on the TER effect [21] , [22] , [23] , [24] , [25] , [26] , [27] , [28] , [29] , [30] , [31] , [32] , [33] . Therefore, it is essential to examine the impact of different electrode materials on the TER characteristics of FTJs. Furthermore, the TER effect associated with ferroelectric switching is inferred from the occurrence of resistance switching at voltages corresponding to the coercive fields of the ferroelectric tunnel barrier. However, as pointed out earlier, this necessary condition is not sufficient to distinguish the ferroelectric-driven TER (FE-TER) from resistance-switching phenomena resulting from—so to speak—‘redox’ reactions [35] . Indeed, given that the very high coercive fields of ultrathin ferroelectric films fall into the electric-field range where the occurrence of a soft breakdown of the film cannot be excluded, there remain concerns that stochastic redox-based resistance switching might be misinterpreted as the FE-TER [36] , [37] , [38] , [39] , [40] , [41] . Therefore, it is of crucial importance to investigate both the TER effect and the redox-based resistive switching in a single FTJ to undoubtedly distinguish between the two different phenomena. In this work, we have fabricated asymmetric FTJs comprising La 0.7 Sr 0.3 MnO 3 (LSMO) bottom electrodes (BEs), 3-nm-thick BTO tunnel barriers and two different top electrodes (Au and Cu TEs). The I–V characteristics of these FTJs are measured by applying a voltage to the micron-sized TEs using a conductive atomic force microscope (C-AFM). The ferroelectric behaviour of the BTO barrier is identified using a piezoresponse force microscopy (PFM) technique. Performing additional capacitance measurements and analysing the complete set of experimental data theoretically, we propose an explanation for the observed giant electrode effect on the TER of the asymmetric FTJs. In addition, we examine the redox-based resistance-switching behaviour in the same FTJs to distinguish it from the TER effect. X-ray diffraction High-quality epitaxial LSMO/BTO heterostructures used in this study were deposited on a (001)-oriented single-crystalline SrTiO 3 (STO) substrate. AFM measurements on the LSMO/BTO heterostructures revealed atomically flat terraces separated by steps of ~0.4 nm height (a single unit cell), which is similar to those of the STO substrate (shown in Fig. 1e ). The X-ray diffraction (XRD) patterns identified that their crystallographic planes were parallel to the (001) planes of STO (see Fig. 1a ), that is, the BTO tetragonal c axis was perpendicular to the substrate surface. To assess the substrate-induced strains and to evaluate the lattice parameters of the heterostructures, X-ray reciprocal space mapping measurement was performed around the asymmetric (103) Bragg reflection. As can be seen from the reciprocal space map shown in Fig. 1b , the LSMO/BTO heterostructures were fully strained in a compressive manner, ensuring a high polarization in the BTO film [16] . The in-plane and perpendicular-to-plane lattice constants of the ultrathin BTO film was found to be 3.905 and 4.134 Å, respectively. 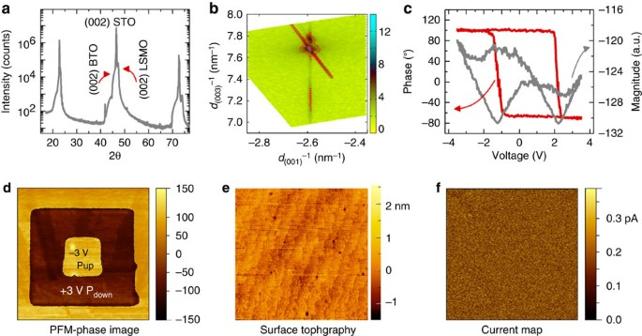Figure 1: XRD and PFM analysis of LSMO/BTO heterostructure. (a) XRD pattern of a LSMO/BTO heterostructure deposited on a (001)-oriented STO single-crystal substrate. (b) Reciprocal space map around the asymmetric (103) Bragg reflection measured on a LSMO (30 nm)/BTO (3 nm) heterostructure. (c) Hysteretic behaviour of the PFM phase and amplitude signals measured on the bare surface of 3-nm-thick BaTiO3film as a function of the bias applied via conducting tip. (d) PFM phase image of the square domains with downward and upward polarizations written with±3 V on the same BaTiO3film. (e) AFM topography image of the surface region (4 × 4 μm2) enclosing the written domains. (f) Electric–current image of the same written domains with downward and upward polarizations. Figure 1: XRD and PFM analysis of LSMO/BTO heterostructure. ( a ) XRD pattern of a LSMO/BTO heterostructure deposited on a (001)-oriented STO single-crystal substrate. ( b ) Reciprocal space map around the asymmetric (103) Bragg reflection measured on a LSMO (30 nm)/BTO (3 nm) heterostructure. ( c ) Hysteretic behaviour of the PFM phase and amplitude signals measured on the bare surface of 3-nm-thick BaTiO 3 film as a function of the bias applied via conducting tip. ( d ) PFM phase image of the square domains with downward and upward polarizations written with±3 V on the same BaTiO 3 film. ( e ) AFM topography image of the surface region (4 × 4 μm 2 ) enclosing the written domains. ( f ) Electric–current image of the same written domains with downward and upward polarizations. Full size image PFM and C-AFM Ferroelectric properties of the BTO film were investigated at room temperature using the PFM. First, we measured the local out-of-plane piezoresponse on the bare surface of the 3-nm-thick BTO film. As shown in Fig. 1c , a clear hysteretic behaviour was observed in both phase (~180° difference) and magnitude signals, acquired at a resonance frequency of the cantilever (542 kHz) as a function of a voltage V applied to the C-AFM tip (the LSMO BE was grounded). These results clearly show ferroelectric switching behaviour of the 3-nm-thick BTO film. The ferroelectric switching (coercive) voltages creating the downward polarization P ↓ (directed towards the LSMO BE) and the upward polarization P ↑ (directed towards the C-AFM tip) were found to be about +2.5 and −1.2 V, respectively. Applying a constant voltage V =±3 V to the tip and scanning the film surface, we poled different regions of the BTO film. Figure 1d shows a PFM phase image of the poled film, acquired at a frequency close to the cantilever resonance frequency. As the ultrathin BTO film was subjected to a high in-plane biaxial compressive strain of ~2%, ensuring perpendicular-to-plane polarization orientations [20] , a large phase contrast of ~180° between the square domains written at +3 and −3 V qualitatively demonstrates the appearance of the P ↓ and P ↑ states, respectively. The unpoled region outside the larger domain displays the out-of-plane spontaneous polarization P ↑ , which can be attributed to the presence of substrate-induced strains and internal bias in the BTO film. The topography image acquired during the PFM phase image acquisition indicates no surface deformation during the film poling (see Fig. 1e ). Interestingly, no change in the local conductance of the BTO film after the polarization switching was observed, as can be seen in the current map shown in Fig. 1f . This finding is not consistent with the previous observations [23] . We believe that it was due to the very low leakage current of the BTO barrier (see Figs 2b and 3b ) and the high contact resistance between the tip and the BTO surface, which reduce the current below the measurement sensitivity of our instrument (~1 pA). 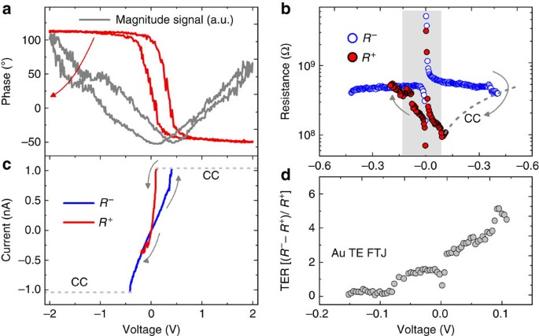Figure 2: TER effect in LSMO/BTO/Au FTJ. (a) Hysteretic behaviour of the PFM phase and magnitude signals plotted as a function of the bias voltage applied to the Au TE of the LSMO/BTO/Au FTJ. (b) A typicalI–Vcurve and (c) the correspondingR–Vbehaviour (CC denotes compliance current). (d) Bias dependence of TER derived from theR–Vcharacteristics in the shadowed voltage range. All measurements were performed at room temperature using C-AFM. Figure 2: TER effect in LSMO/BTO/Au FTJ. ( a ) Hysteretic behaviour of the PFM phase and magnitude signals plotted as a function of the bias voltage applied to the Au TE of the LSMO/BTO/Au FTJ. ( b ) A typical I–V curve and ( c ) the corresponding R–V behaviour (CC denotes compliance current). ( d ) Bias dependence of TER derived from the R–V characteristics in the shadowed voltage range. All measurements were performed at room temperature using C-AFM. 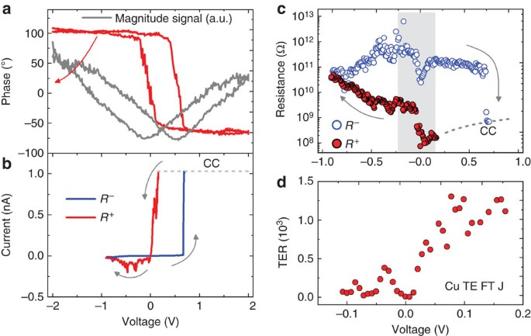Figure 3: TER effect in LSMO/BTO/Cu FTJ. (a) Representative PFM phase and magnitude signals obtained on the LSMO/BTO/Cu FTJ. (b) A typicalI–Vand (c) the correspondingR–Vcharacteristics of the same FTJ. (d) Bias dependence of TER derived from theR–Vcharacteristics in the shadowed voltage range. Full size image Figure 3: TER effect in LSMO/BTO/Cu FTJ. ( a ) Representative PFM phase and magnitude signals obtained on the LSMO/BTO/Cu FTJ. ( b ) A typical I–V and ( c ) the corresponding R–V characteristics of the same FTJ. ( d ) Bias dependence of TER derived from the R–V characteristics in the shadowed voltage range. Full size image Observation of giant electrode effect on TER Next, we studied ferroelectric properties of the BTO barriers sandwiched between two electrodes in complete FTJs. The latter were fabricated by covering the 3-nm-thick BTO film grown on LSMO by Au and Cu TEs of 2 μm 2 areas and PFM measurements were performed with the C-AFM tip brought into contact with the TE. Figures 2a and 3a show the phase and amplitude of the local out-of-plane piezoresponse for the FTJs with Au and Cu TEs, respectively. The observed reproducible phase change ~180° of the piezoresponse during the voltage sweep indicates that the BTO film retains its ferroelectric state in the presence of the TE as well. It should be noted that extended TEs minimize the electrostatic contribution to the PFM signal and make the electric field inside the probed film almost homogeneous [42] . Therefore, significant differences in coercive voltages between the cases of the bare BTO film under direct tip-BTO contact ( Fig. 1c ) and the TE-covered BTO film ( Figs 2a and 3a ) are expectable. The coercive voltages of the TE-covered BTO barrier, determined from the minima in the piezoresponse amplitude, were found to exhibit distributions in the ranges V down ≈0.3−0.8 V for the P ↑ → P ↓ switching and V up ≈−0.25−0.2 V for the P ↓ → P ↑ one. Hence, the mean coercive field E c =| V down — V up |/2 t of the BTO film with the thickness t =3 nm ranges from 0.6 to 1 MV cm −1 . These values are consistent with the coercive fields reported for very thin ( t ~5 nm) BTO films earlier [17] , [43] , [44] . This result is a strong indication of the good quality of the fabricated ultrathin BTO barrier. To investigate TER effect, the same FTJs were further characterized by measuring their hysteretic I–V curves. To that end, quasi-static voltage sweeps with a sweep rate of 0.05 Vs −1 were applied to the Au and Cu TEs via the C-AFM tip. The BE was grounded and a compliance current of 1 nA was set during the measurements to avoid soft dielectric breakdown of the junctions. Representative I–V curves and the corresponding resistance–voltage ( R – V ) ones are shown in Fig. 2 (FTJ with Au TE) and Fig. 3 (FTJ with Cu TE) (we take R = V / I ). Unlike the LSMO/BTO/tip junction, the FTJs with the extended TEs display hysteretic I–V behaviour characterized by two dissimilar resistances R − and R + . Although these resistances vary significantly with the applied voltage, the existence of the distinct high- and low-resistance states of the FTJs is evident. It should be noted that the initial high-resistance state (HRS with R = R − ) switches to the low-resistance state (LRS with R = R + ) at a certain positive voltage and recovers during the negative voltage sweep. The revealed hysteretic electrical behaviour and the occurrence of resistive switching events at the coercive voltages of the BTO barrier (compare panels a and b in Figs 2 and 3 ) point to the FE-TER effect. Importantly, these features were found to be reproducible during 20 cycles of voltage sweeps. The apparent FE-TER effect was quantified by the TER ratio ( R − — R + )/ R + , plotted as a function of the applied voltage in Figs 2d and 3d . It is seen that, for both FTJs (with Au and Cu TEs), the observed TER ratios increase monotonically with increasing voltage, not showing any maximum at zero bias. As the setting of compliance current is required for non-destructive electrical measurements of the FTJs, the TER ratio cannot be evaluated in the whole voltage range. Although the FTJs with Au and Cu TEs display qualitatively similar FE-TER behaviours, their TER ratios differ dramatically. Indeed, Figs 2d and 3d show that the TER ratio of the LSMO/BTO/Au FTJ varies from 2 at V =50 mV to about 5 at V ≈0.15 V, whereas the LSMO/BTO/Cu FTJ shows a TER of ~1,000 at V =0.1−0.15 V. Thus, the TER ratios of the two FTJs may differ by more than two orders of magnitude at the same voltage. This drastic difference demonstrates the giant electrode effect on TER, which is additionally supported by the absence of measurable resistive switching in the LSMO/BTO/tip junctions on polarization reversal (see Fig. 1f ). Origin of giant electrode effect in asymmetric FTJs Let us attempt now to find a reasonable physical explanation for the revealed giant electrode effect on the FE-TER and its voltage dependence. The TER exhibited by the asymmetric FTJs may be attributed to (i) the depolarizing-field effect [12] , [13] or/and (ii) the microscopic interfacial effect [12] , [45] . Up to now, theoretical studies of these effects have been mostly focused on the resulting TER ratios at zero voltage, because the two opposite remanent polarization states are expected to be equally stable at V =0 (that is, V up =− V down ). This is true, however, only in the absence of an internal electric field in the tunnel barrier, which may be caused, for instance, by a difference in the work functions between TE and BE [46] , [47] . As this internal electric field shifts the centre of the polarization-voltage hysteresis loop from V =0 to a particular finite voltage, the representative TER ratio is no longer expected at zero voltage. This feature should be taken into account in the theoretical description of our asymmetric FTJs, where the internal electric field appears to be significant (see Figs 2a and 3a ). To describe the dependence of the TER on the applied voltage, one can use the model of a trapezoidal barrier [47] . This model renders possible to calculate the density of tunnel current J=I / A as a function of voltage V using the barrier heights φ 1 and φ 2 at the two ferroelectric–electrode interfaces, barrier thickness t , electron charge e and effective mass m b of tunnelling charge carriers in the barrier as input parameters. For barriers with a thickness and voltages satisfying the inequality | eV |/2<min { φ 1 , φ 2 }, the following analytical relation has been derived: [48] where and ħ is the reduced Planck constant. Using equation (1), one can find the FTJ’s conductance G = J A / V and resistance R =1/ G , which may depend on the polarization orientation in the barrier owing to related changes in φ 1 and φ 2 . When these changes are dominated by the depolarizing-field effect, from the electrostatic considerations we obtain where and are the barrier heights in the absence of ferroelectric polarization, P 3 = P 3 ( t ) is the thickness-dependent equilibrium out-of-plane polarization in the barrier, c m1 and c m2 are the capacitances of screening space charges (per unit area) in dissimilar TE and BE, and is the total interfacial capacitance. Equation (2) shows that the mean barrier height changes by the amount after the polarization reversal, which gives rise to the TER effect in asymmetric FTJs. The microscopic interfacial effect on the barrier profile results from the ferroelectric shifts of ions at two barrier–electrode interfaces [12] . Therefore, we can describe it phenomenologically via the relations and . In asymmetric FTJs involving two dissimilar electrodes, ξ 1 ≠ ξ 2 so that the polarization reversal again changes the mean barrier height, thus producing TER. In general, both the depolarizing-field and microscopic interfacial effects influence the barrier heights at the two ferroelectric–electrode interfaces considerably. In the first approximation, this joint influence can be quantified by the relationships and . These formulae indicate that it is rather difficult to separate two contributions to the TER effect via an analysis of experimental data. Furthermore, as the capacitance measurements provide information on the total interfacial capacitance only (see below), additional symmetric samples with identical electrodes are needed to determine c m1 and c m2 . On the other hand, first-principles calculations render possible to evaluate the depolarizing-field and microscopic interfacial effects on TER separately [45] . When variations of φ 1 and φ 2 with voltage are negligible, the resistance R ( V ) of an asymmetric junction shows a parabolic-like behaviour with a maximum located at some non-zero voltage V m (see Fig. 4a ). As a result, the TER ratio may change with voltage significantly, exhibiting a monotonic increase for the considered representative FTJ (see Fig. 4b ). Remarkably, the TER ratios of both experimentally studied FTJs display the same general trend ( Figs 2d and 3d ). It should be noted that the observed voltage dependences of the high resistances R − of our junctions ( Figs 2c and 3c ) are mostly similar to the predicted decrease of resistance with increasing difference | V — V m |. At the same time, the low-resistances R + show the opposite behaviour. 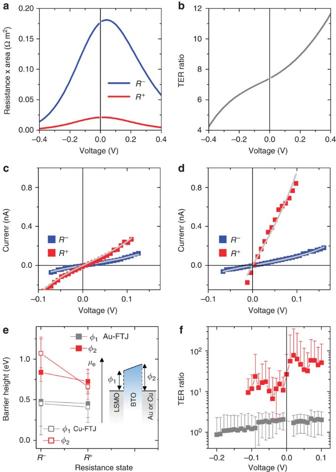Figure 4: Theoretical analysis of TER effect. (a,b) Voltage dependences of FTJ resistances in two polarization states and the TER ratio calculated for a representative junction using the following parameters taken from ref.48:φ1=0.48 eV,φ2=0.96 eV (R+),φ1=0.24 eV,φ2=1.52 eV (R−) andmbequal to the free electron massme. (c,d) RepresentativeI–Vcurves of the LSMO/BTO/Au and LSMO/BTO/Cu junctions, respectively, and their fitting by equation (1) (grey lines). (e) Statistical data on the barrier heightsφ1andφ2determined by fitting theI–Vcurves of FTJs with Au and Cu TEs measured on five different junctions of the same area (2 μm2) for each FTJ type (the inset depicts a schematic profile of electron’s electrochemical potentialμeacross the junction). (f) Statistical data on the TER ratios of FTJs with Au and Cu TEs obtained from the same five junctions for each FTJ type. Figure 4: Theoretical analysis of TER effect. ( a , b ) Voltage dependences of FTJ resistances in two polarization states and the TER ratio calculated for a representative junction using the following parameters taken from ref. 48 : φ 1 =0.48 eV, φ 2 =0.96 eV ( R + ), φ 1 =0.24 eV, φ 2 =1.52 eV ( R − ) and m b equal to the free electron mass m e . ( c , d ) Representative I–V curves of the LSMO/BTO/Au and LSMO/BTO/Cu junctions, respectively, and their fitting by equation (1) (grey lines). ( e ) Statistical data on the barrier heights φ 1 and φ 2 determined by fitting the I–V curves of FTJs with Au and Cu TEs measured on five different junctions of the same area (2 μm 2 ) for each FTJ type (the inset depicts a schematic profile of electron’s electrochemical potential μ e across the junction). ( f ) Statistical data on the TER ratios of FTJs with Au and Cu TEs obtained from the same five junctions for each FTJ type. Full size image The voltage-independent barrier heights, however, are not characteristic of FTJs. Indeed, φ 1 and φ 2 should vary owing to the dependence of polarization P 3 on the electric field E 3 in the ferroelectric barrier. In addition, the lattice strains of piezoelectric origin change the position of the conduction-band edge [12] , which may modify φ 1 and φ 2 significantly. These peculiarities of FTJs could alter the dependence R ( V ) when the barrier height at V =0 is small, as it is expected for the LRS ( R = R + ). The influence of piezoelectric strains on the barrier thickness t and the electron effective mass m b may complicate the voltage dependence of junction’s resistance and TER additionally [12] . To clarify whether the observed giant electrode effect on TER may be caused by the influence of the TE on the depolarizing field in the tunnel barrier, we measured the capacitance densities c of LSMO/BTO/Cu and LSMO/BTO/Au heterostructures as a function of the BTO thickness t (see Fig. 5 ). As the reciprocal capacitance c −1 linearly depends on t , it is possible to determine the interfacial capacitances c i of the two heterostructures. Extrapolating c −1 ( t ) to zero thickness, we found that and . These relations indicate that the capacitance of the BTO/Cu interface is smaller than that of the BTO/Au one, that is, c Cu < c Au . At the same time, the positive voltage sweep applied to the Cu or Au TE results in a jump from the HRS to the LRS (see Figs 2b and 3b ). To explain this type of ferroelectric resistive switching by the depolarizing-field effect, it is necessary to assume that the capacitance of the LSMO/BTO interface is smaller than those of the BTO/Cu and BTO/Au ones [12] . Using this additional requirement, we obtain the inequality c LSMO < c Cu < c Au , which can be rewritten in the form . Hence, the magnitude of the depolarizing-field-induced change in the mean barrier height after the polarization reversal is expected to be larger in the LSMO/BTO/Au junction than in the LSMO/BTO/Cu one. As the TER is mostly governed by , we arrive at the conclusion that the depolarizing-field effect would lead to an increase in the TER ratio after the replacement of the Cu TE by the Au one. This conclusion, which is supported by an accurate analysis based on equations (1) and (2), is opposite to the observations. Owing to this contradiction, we can probably rule out that TE-induced changes in the depolarizing field are responsible for the giant electrode effect on TER observed in our FTJs. 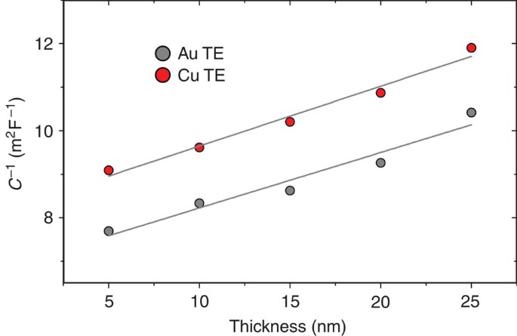Figure 5: Determination of interfacial capacitances of LSMO/BTO/Au(Cu) junctions. Thickness dependence of the reciprocal capacitance density obtained for LSMO/BTO-based ferroelectric capacitors with 2,500-μm2-sized Au and Cu TEs. The straight lines are linear fits to the experimental data. Figure 5: Determination of interfacial capacitances of LSMO/BTO/Au(Cu) junctions. Thickness dependence of the reciprocal capacitance density obtained for LSMO/BTO-based ferroelectric capacitors with 2,500-μm 2 -sized Au and Cu TEs. The straight lines are linear fits to the experimental data. Full size image Therefore, the revealed large difference in the TER ratio between the LSMO/BTO/Cu and the LSMO/BTO/Au FTJs should be attributed to the microscopic interfacial effect. To demonstrate the feasibility of this explanation, we fitted the measured I–V curves in the range of small voltages using equation (1). The barrier heights φ 1 and φ 2 were regarded as adjustable parameters independent of applied voltage in the considered voltage range and the effective mass m b was assumed to be equal to the free electron mass m e (ref. 48 ). As is seen from Fig. 4c,d , the I–V curves of both FTJs can be fitted by equation (1) with a good accuracy for both resistance states. The barrier heights, determined by the method of least squares, have the following values: φ 1 =0.26 eV, φ 2 =0.78 eV ( R + ) and φ 1 =0.24 eV, φ 2 =0.92 eV ( R − ) for the LSMO/BTO/Au FTJ and φ 1 =0.30 eV, φ 2 =0.61 eV ( R + ) and φ 1 =0.37 eV, φ 2 =0.76 eV ( R − ) for the LSMO/BTO/Cu FTJ. These barrier heights are similar to those obtained by Gruverman et al . [48] for SrRuO 3 /BTO/Pt junctions. To obtain statistical data on variations in the barrier heights from junction to junction and from cycle to cycle, the fitting procedure was repeated for five different FTJs of each type (with the same area of 2 μm 2 ) and for five I–V cycles for each junction on average. The obtained results, which are summarized in Fig. 4e , demonstrate that despite considerable variations in the values of φ 1 and φ 2 , all barrier heights have reasonable magnitudes ~0.25−1 eV. Interestingly, the change Δ φ 2 in the barrier height φ 2 at the BTO/Au(Cu) interface on switching between R + and R − appears to be much larger in the case of the Cu TE. In contrast, only small changes in the barrier height φ 1 at the LSMO/BTO interface take place after resistive switching. As the TER ratio is governed by changes in the barrier heights, the giant electrode effect on TER may be attributed to the difference in Δ φ 2 between the junctions with Cu and Au TEs. Importantly, all five studied FTJs with the Cu TE have much higher TER ratios than five junctions with the Au TE (see Fig. 4f ). Hence, the revealed giant electrode effect has a high reproducibility. Typical I–V curves of the FTJs under evaluation are shown in Supplementary Fig. 1 . It should be emphasized that a careful FTJ design is required to guarantee strong FE-TER effect. The theoretical calculations predict that the change in the mean barrier height, resulting from the polarization reversal, is directly proportional to the average out-of-plane polarization ‹ P 3 › in the ferroelectric interlayer. Hence, appropriate electromechanical conditions that enhance ‹ P 3 › have to be created in this layer. In particular, the choice of electrode materials should provide sufficiently large total interfacial capacitance , while the substrate used for the device fabrication has to create high compressive in-plane strains reducing the detrimental influence of the depolarizing field on ‹ P 3 › [20] . At the same time, the numerical estimates based on the typical values of polarization of ultrathin BTO films ( P 3 ~0.3 Ccm −2 ) [16] and the difference between reciprocal space-charge capacitances of electrodes made of elemental metals and conductive oxides ( ) [20] , [49] show that the depolarizing-field effect is expected to give a considerable contribution to the TER of FTJs involving the BTO barrier ( ~0.3−0.5 eV). Accordingly, the microscopic interfacial effect on TER in our FTJs appears to be strong enough to override the depolarizing-field one and the coexistence of these two effects should be taken into account in the design of FTJs. Finally, the build-in electric field usually existing in asymmetric FTJs influences their TER as well. When this field exceeds the respective coercive field of a ferroelectric barrier, the TER effect is not present at zero voltage anymore. Although the build-in field can be compensated by an external field created by the applied bias V , it still influences the TER ratio at a given voltage. As can be seen from Figs 2d and 3d , in our FTJs the TER ratio is rather small at V =0. Therefore, sufficient bias voltage is needed to achieve a strong resistance change after the polarization reversal, which is required for the memory applications of FTJs. Area dependence of giant electrode effect The giant electrode effect discussed so far was observed for FTJs with the 2 μm 2 area. To indentify probable dependence of this effect on the junction’s area, we studied the I–V behaviour of additional FTJs of three different areas (45, 400 and 2,500 μm 2 ). Four junctions of each area have been investigated to evaluate junction-to-junction variations in the electrical properties. 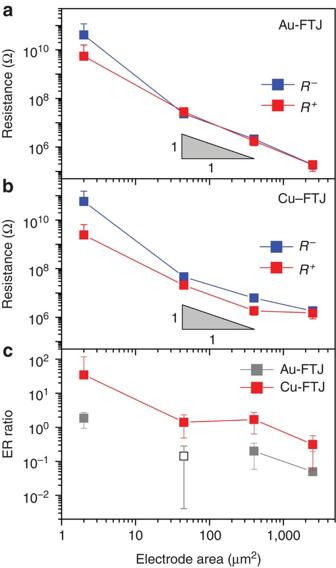Figure 6: Area dependence of electroresistance effect. ResistancesR−andR+measured at a voltage of 0.05 V during the upward and downward voltage sweeps for FTJs with (a) Au (b) and Cu TEs of different areas (2, 45, 400 and 2,500 μm2) and (c) the corresponding electroresistance ratio (R−—R+)/R+. The grey triangles point to a slope of unity. Note that the mean ER ratio of the FTJ with 45-μm2-sized Au TE was seemingly negative; it is separately plotted incby using an open square. Figure 6 summarizes the experimental results obtained for the resistances R − and R + measured at a voltage of 0.05 V during the upward and downward voltage sweeps and the corresponding electroresistance (ER) ratio ( R − — R + )/ R + . It is seen that both resistances decrease rapidly with increasing electrode area and the FTJs with the 2 μm 2 area have higher resistances than expected from the extrapolation of the results obtained for larger FTJs. Furthermore, the ER ratio strongly reduces with increasing electrode area for FTJs of both studied types and even changes sign for some junctions with the Au TE (see Fig. 6c ). Figure 6: Area dependence of electroresistance effect. Resistances R − and R + measured at a voltage of 0.05 V during the upward and downward voltage sweeps for FTJs with ( a ) Au ( b ) and Cu TEs of different areas (2, 45, 400 and 2,500 μm 2 ) and ( c ) the corresponding electroresistance ratio ( R − — R + )/ R + . The grey triangles point to a slope of unity. Note that the mean ER ratio of the FTJ with 45-μm 2 -sized Au TE was seemingly negative; it is separately plotted in c by using an open square. Full size image These observations most probably imply the presence of another transport mechanism in our FTJs, which acts in parallel to the electron tunnelling and becomes more important in junctions with large areas. This mechanism may be attributed to imperfections in the BTO film, such as etch pits, voids, dislocations and foreign particles (see Fig. 1e ), which might be introduced randomly during the substrate treatment or film growth. The presence of such imperfections, probably serving as local conduction paths, is much more probable in larger FTJs. Hence, the electric current flowing through such imperfections should increase with the junction’s area and, in FTJs with large areas, may become even stronger than the current caused by electron tunnelling. In view of the probable presence of another transport mechanism, we used the term ‘electroresistance’ instead of TER in this section. Redox-based resistance switching Although the occurrence of the resistive switching in our FTJs at the coercive voltages of the BTO barrier indicates its ferroelectric origin, BTO is also known as a redox-based resistance-switching material [35] . Therefore, it is critically important to investigate the redox-based resistive switching behaviour of our FTJs to clearly distinguish this mechanism from the FE-TER effect. It is known that an electroforming process is usually required to activate redox-based resistance-switching phenomena in complex oxide materials [50] . Electroforming is generally achieved by applying high electric fields that can lead to soft breakdown of the insulating oxide layer. Such fields induce the formation of localized (filamentary), defect-rich and structurally/chemically altered regions that have much higher electrical conductivity than the surrounding insulating matrix. It can be assumed that redox-based resistance-switching effects result from physical/chemical phase transformations occurring somewhere along these defective, conducting filamentary paths, which can be brought forth by, for example, local Joule heating in combination with significant redistributions of mobile ionic species under electric field action [50] . In the present study, considering the electric fields required to trigger a soft breakdown of the BTO tunnel barrier, we applied comparatively large-range quasi-static voltage sweeps (starting from maximum negative voltage) to the LSMO/BTO/Au and LSMO/BTO/Cu heterostructures using the C-AFM tip to contact the TEs. 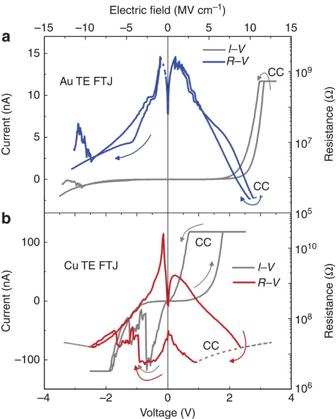Figure 7: Redox-based resistance switching. Typical redox-based resistance switching characteristics (I–VandR–V) of LSMO/BTO heterostructures with (a) Au and (b) Cu TEs. In both panels, the grey curve shows anI–Vcharacteristic. The blue and red curves demonstrateR–Vcharacteristics of the FTJs with Au and Cu TEs, respectively. CC, compliance current. The upper horizontal axis shows the electric field in the tunnel barrier, which corresponds to the applied voltage given by the lower horizontal axis. Figure 7 shows the measured I–V and corresponding R–V characteristics for the redox-based resistance switching of the LSMO/BTO/Au and the LSMO/BTO/Cu junctions. One can clearly see that in this case the voltages required for the switching to the LRS and back to the HRS are five to ten times higher than the average switching voltages of the FE-TER effect. Accordingly, the electric fields required for the redox-based switching ( ca . 4−8 MV cm −1 ) appear to be much higher than the ferroelectric coercive field of the studied BTO layer. This drastic difference may be attributed to high activation energies of the microscopic processes governing the redox-based resistive switching, such as the field-induced migration/re-distributions of anions and/or cations in oxide materials [39] , [50] , [51] . These energies probably exceed considerably the activation energy of ferroelectric domain nucleation at electric fields approaching the coercive field of our ultrathin BTO layer. Figure 7: Redox-based resistance switching. Typical redox-based resistance switching characteristics ( I–V and R–V ) of LSMO/BTO heterostructures with ( a ) Au and ( b ) Cu TEs. In both panels, the grey curve shows an I–V characteristic. The blue and red curves demonstrate R–V characteristics of the FTJs with Au and Cu TEs, respectively. CC, compliance current. The upper horizontal axis shows the electric field in the tunnel barrier, which corresponds to the applied voltage given by the lower horizontal axis. Full size image We have observed the TER effect in FTJs comprising an ultrathin BTO barrier epitaxially grown on a LSMO BE and covered by micron-sized Au and Cu TEs. Combining the I–V measurements performed by C-AFM with the PFM characterization, we found that the resistance switching occurred at voltages consistent with the coercive voltages of the BTO barrier, which confirms its ferroelectric origin. Remarkably, the giant electrode effect on the TER was revealed, which manifests itself in a drastic reduction (by two orders of magnitude) of the relative resistance changes on polarization reversal when the Cu TE is replaced by the Au one. A theoretical analysis of the I–V curves allowing for the results of additional capacitance measurements indicates that the observed resistance switching is caused by the microscopic interfacial effect, but not by the depolarizing field one. We also found that the TER effect becomes undetectable when the conducting AFM tip is employed as a TE. This feature may be attributed to a strong suppression of the tunnel current by an additional local potential barrier formed at the BTO-tip joint, which is very probable for the AFM tip brought into ‘loose’ contact with the ferroelectric film using an applied mechanical force. At the same time, the barrier height at the epitaxial BTO/BE interface, where the contacting materials are bound by strong interatomic forces, should still change after the polarization reversal owing to the microscopic and depolarizing-field effects. Hence, under favourable contact conditions the TER effect can be observed even in FTJs where the conducting AFM tip is used as a TE [23] , [48] . It should be emphasized that it is very unlikely that the TER effect in our FTJs is governed by structural defects. As the ultrathin epitaxial BTO film is fully strained by the STO substrate, misfit dislocations should be practically absent here. Ferroelastic domain walls also cannot form in the BTO film, because the substrate-induced high (~2%) compressive in-plane strains strongly favour the single-domain state [43] . The transmission electron microscope images of the BTO/LSMO interface available in the literature demonstrate the sharpness of this interface [22] , which points to the absence of a defect-rich layer at the BTO/BE interface. Of course, the formation of an intermediate layer at the BTO/TE interface cannot be ruled out a priori . Given that Cu is electrochemically more active than Au, it is more likely to be that junctions with the Cu TE contain CuO x interfacial layers, which are either insulating or semiconducting depending on their stoichiometry. As CuO x is known as a redox-based resistive-switching material [50] , it could give rise to electric-field-induced resistance changes in the LSMO/BTO/Cu junction. However, our scanning transmission electron microscopy (STEM) analysis of the LSMO/BTO/Cu junction clearly demonstrates the absence of such a CuO x interlayer. Indeed, the cross-sectional STEM image and distributional profiles of Cu and O atoms across the junction, shown in Fig. 8a , provide no evidence on the interlayer formation. In addition, the electron energy loss spectroscopy shows that the electron energy loss spectra of Cu in the vicinity of the BTO/Cu interface are clearly of metallic Cu rather than any CuO x , as can be seen in Fig. 8b . Thus, the formation of CuO x and its effect on the FE-TER can be excluded. It should be emphasized that our experimental results are fully consistent with this microscopic observation. For instance, if the CuO x layer were present in the junction, this layer should manifest itself in a strong decrease in the junction’s interfacial capacitance, which is hardly consistent with the fact that the measured interfacial capacitance densities of LSMO/BTO/Cu and LSMO/BTO/Au junctions differ only slightly (0.12 versus 0.14 F m −2 ). Moreover, the mechanism of resistive switching associated with the CuO x layer is inconsistent with our observations for the following two reasons. First, the redox-based resistive switching is generally initiated by electroforming process that introduces either oxygen vacancies or sub-oxide phase(s) in hypo-stoichiometric transition metal oxides such as BTO [50] . However, no electroforming was required for the observed FE-TER effect. Second, if CuO x were involved in the resistance switching in our junctions, the transition from the HRS to the LRS would take place when a negative, rather than positive, voltage is applied to the Cu TE. Indeed, the application of a positive voltage to the Cu TE would oxidize Cu at the interface (anodization of Cu), which would consequently lead to an increase in the junction’s resistance as CuO x is much more resistive than Cu. On the contrary, the observed jump from the HRS to the LRS occurs at a positive voltage applied to the Cu or Au TE (see Figs 2b and 3b ). 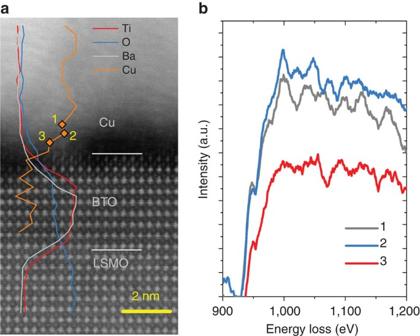Figure 8: STEM analysis on LSMO/BTO/Cu FTJ. (a) Cross-sectional STEM image of the LSMO/BTO/Cu FTJ and distributional profiles of Ti, O, Ba and Cu across the junction. (b) Electron energy loss spectroscopy spectra of Cu in the vicinity of the BTO/Cu interface at three locations, numbered 1, 2 and 3 ina. Figure 8: STEM analysis on LSMO/BTO/Cu FTJ. ( a ) Cross-sectional STEM image of the LSMO/BTO/Cu FTJ and distributional profiles of Ti, O, Ba and Cu across the junction. ( b ) Electron energy loss spectroscopy spectra of Cu in the vicinity of the BTO/Cu interface at three locations, numbered 1, 2 and 3 in a . Full size image As the presence of a CuO x interfacial layer in the LSMO/BTO/Cu junction can be ruled out, the Cu TE hardly works as a sink for oxygen ions and a source of oxygen vacancies in the adjoining BTO layer. As a result, the density of oxygen vacancies, which are apparently present in this perovskite layer [52] , [53] despite our attempts to suppress their formation here during the fabrication process (see Methods), is expected to be the same in both studied FTJs. Hence, the observed giant electrode effect on TER cannot be attributed to the motion of oxygen vacancies across the junction as well. Finally, it should be noted that the revealed emergence of the FE-TER effect at electric fields much lower than the fields required for the redox-based resistive switching is expected to take place at low temperatures as well. Indeed, the recent experimental study of the BTO/LSMO FTJs showed that the switching fields characteristic of the FE-TER effect stay constant below 250 K [54] , whereas the electric fields necessary for the redox-based resistive switching generally increase significantly at low temperatures [55] . Therefore, the difference between two discussed switching fields should become even larger with lowering the temperature. Further studies, focusing on the temperature dependence of switching voltages and ‘time-to-switch’ analysis at constant bias, could shed light on the kinetics of the FE-TER and redox-reaction-based resistance-switching phenomena [32] . Sample preparation The high-quality epitaxial LSMO/BTO heterostructure used in this study was deposited on a (001)-oriented STO single-crystal substrate. The surface of the commercially obtained substrate was chemically etched with buffered hydrofluoric acid solution for 30 s and then annealed at 875 °C under an oxygen pressure of 0.14 mbar to achieve Ti-O-terminated surface. The LSMO(30 nm)/BTO(3 nm) heterostructure was grown via pulsed laser deposition at a substrate temperature of 700 °C in a 0.14-mbar pure oxygen atmosphere. After deposition, the sample was cooled down to room temperature under an oxygen pressure of 75 mbar to suppress oxygen vacancy formation in the film. Au and Cu TEs of thicknesses 5–6 nm were deposited onto the BTO film by thermal evaporation. The TEs were patterned using a stencil mask, whose areas are in the 2–2,500 μm 2 range. The Cu TEs were covered with an in situ formed ~4-nm-thick Au layer to avoid their oxidation by atmospheric oxygen molecules. Note that both types of TEs shared the same BTO film so that possible variations of the microscopic properties of LSMO and BTO were minimized. In addition, the sample was heated up to 120 °C before the TE deposition to remove the water molecules from the surface. XRD and PFM characterization The crystal structure of the epitaxial layers was characterized by means of XRD and reciprocal space mapping using a Seifert Space XRD 4-circle diffractometer system. PFM measurements were performed at room temperature using an AIST-NT SPM instrument. Commercially available Pt-coated silicon tips were employed for the PFM measurements at typical contact resonance frequencies of 0.5–0.6 MHz. I–V measurements The I–V measurements of FTJs with 2 μm 2 TE area were performed using a C-AFM tip by applying quasi-static voltage sweeps to the Au or Cu TE, while the BE was grounded. An Agilent 33220A waveform generator and a Keithley 6517 electrometer resistance system were used in the I–V characterization of the FTJs with large TE areas (45, 400 and 2,500 μm 2 ). Capacitance–voltage measurements To evaluate the interfacial capacitance for both types of FTJs, capacitance versus voltage measurements were done using a precision HP4284A LCR meter. The measurements were performed at room temperature using a small sinusoidal signal of 5 mV (peak-to-peak) at 10 kHz and a voltage sweep rate of 5 mV s −1 . The interfacial capacitance was estimated via the extrapolation procedure using the maxima of capacitance–voltage hysteresis loops obtained for five different BTO thicknesses (5, 10, 15, 20 and 25 nm). STEM characterization Microstructural and chemical analysis at the atomic scale was conducted by using a Titan transmission electron microscope at electron acceleration energy of 300 keV. How to cite this article : Soni, R. et al . Giant electrode effect on tunnelling electroresistance in ferroelectric tunnel junctions. Nat. Commun. 5:5414 doi: 10.1038/ncomms6414 (2014).